Supercooled liquids with enhanced orientational order The nature of the glass transition, the transformation of a liquid into a disordered solid, still remains one of the most intriguing unsolved problems in materials science. Recent models rationalize crucial features of vitrification with the presence of medium-range ordered regions coexisting with the isotropic liquid. Here, in line with this prediction, we report an extraordinary enhancement in bond orientational order in ultrathin films of supercooled polyols, grown by physical vapour deposition. By varying the deposition conditions and the molecular size, we could tune the kinetic stability of the liquid phase enriched in bond orientational order towards conversion into the ordinary liquid phase. We observed a strong increase in the dielectric strength with respect to the ordinary supercooled liquid and slower structural dynamics, suggesting the existence of a metastable liquid phase with improved orientational correlations. Isotropic liquids are characterized by the absence of any long-range positional order. Operationally, they are distinguished from solids on the basis of their mechanical response as expressed by the structural relaxation time, τ , defined via Maxwell’s relation [1] as the ratio between the shear viscosity η and the instantaneous shear modulus G ∞ . Materials in which τ is shorter than the experimental observation time are considered liquids, whereas in the opposite case, they are regarded as (disordered) solids. Upon cooling or pressurizing, liquids can transform into the solid state. Depending on their energy landscape and on the thermodynamic and kinetic path they follow, they acquire a periodic structure with full translational order (crystals) or maintain a morphology lacking in long-range order (glasses) [2] , [3] , [4] , [5] . The structural relaxation time increases upon cooling, and the glassy state is achieved when τ exceeds the experimental observation time; upon quenching, this condition occurs at the glass transition temperature, T g . Glasses are thus systems that are out of thermodynamic equilibrium. Although these materials are commonly regarded as disordered systems, crucial features of the glass transition, such as the increase in heterogeneity and the larger cooperativity of the liquid dynamics approaching solidification [6] , [7] , [8] , [9] , can be rationalized by the presence of medium-range ordered regions (MRO) in the liquid phase. Frustration models [10] , [11] , [12] , developed in the past few decades, ascribe this behaviour to the presence of icosahedra, locally preferred structures (LPSs) present in the isotropic liquid at temperatures below the melting point, T m . The formation of these solid-like clusters is driven by maximizing the number of directional bonds that lock the system to local minima in the free-energy landscape. As a consequence, LPSs are metastable, long-lived structures, showing bond orientational order (BOO) while lacking the long-range topological order of the crystal. At low pressures, icosahedra are energetically favoured with respect to clusters with crystallographic symmetry, and the resulting geometric frustration prevents the development of long-range order. In contrast, the two-order parameter model [13] predicts that the frustration of crystallization is due to both kinetic and energetic factors: the presence of an anisotropic potential of intermolecular interaction generates LPSs, whose spatial symmetry is not compatible with the structure of the equilibrium crystal. According both to the paradigm of the frustration models and to the two-order parameter model, supercooled liquids consist of a heterogeneous mosaic of MRO regions, grown in proximity to LPSs and surrounded by the isotropic ordinary liquid (OL). Evidence of such structures has been found in metallic glass formers [14] , [15] , [16] , where the presence of quasi-crystalline clusters with a few topological defects has been detected by diffraction techniques, such as atomic-scale high-resolution transmission electron microscopy and by X-ray, neutron and electron diffraction. An enhanced degree of topological order may be achieved via structural rearrangements, either by annealing below the glass transition temperature (physical aging) [17] or pressurizing [18] , which permits the nucleation of MRO regions in proximity to the quasi-crystalline clusters and the consecutive propagation of a similarly ordered structure. For some metallic glasses, this approach has allowed access to smaller, pre-existing crystalline structures, otherwise undetectable by the aforementioned experimental techniques because the structure factor of an amorphous phase containing topological order is virtually undistinguishable from the structure factor of a glass where molecules are randomly distributed [19] . A method used to grow extended ordered regions is physical vapour deposition (PVD), which has been successfully employed to produce a large family of inorganic misfit layers [20] (where the basic periodicities of one or two interpenetrating layers do not coincide), which are otherwise impossible to obtain. A successive annealing step locks the system into local free-energy minima, dictated by the precursor obtained by PVD. Similarly, PVD of organic glass formers below T g might yield ultradense glasses with highly efficient molecular packing, approaching the limit of the crystal [21] , [22] . Those new materials are characterized by an extremely low excess enthalpy and by a thermodynamic and kinetic stability neither achievable in ordinary glasses, nor by physical aging, hence the name ‘ultrastable glasses’. In contrast to approaching the glass transition by quenching or pressurizing the liquid, vapour deposition in the glassy state operates in thermodynamic equilibrium, taking advantage of the enhanced molecular mobility at the free surface [23] , where evaporated molecules can rapidly sample the energetic landscape and reach deeper minima before being buried by the upcoming layers. This preparation method thus proves to be, at present, the most efficient way to produce glasses with the lowest thermodynamic excess quantities (enthalpy, volume, entropy) [24] . In this report, we present a new method to extend the investigation of medium-range order to organic glass-forming materials by the molecular beam deposition of polyols in the glassy state, followed by annealing in the liquid state. The severe changes in the dielectric permittivity of samples prepared via our method is consistent with an enrichment of the isotropic liquid in long-living MRO regions. Experimental approach to assessing hidden orientational order We exploited the improved sampling of the energy landscape to obtain a liquid phase enriched in regions with medium-range order, following an approach analogous to that introduced to produce misfit layers. We applied this method to prepare ultrathin films of glycerol, threitol and xylitol, glass-forming materials known to form, already in the liquid state, temporary H-bonded networks that rely on highly directional, that is, anisotropic, intermolecular interactions [25] ( E OH···O =8–11 k B T per bond) [26] . This feature, in combination with the improved sampling of the energy landscape, enhances the formation of precursor LPSs located at deep minima. The resulting MRO regions are thus expected to survive long enough to be investigated. The main challenge was the choice of the experimental technique to detect the presence of local order in organic glass-forming systems. In these materials, in contrast to metallic glasses, no evidence of MRO is seen by scattering and diffraction techniques because of the higher degree of freedom, which causes a loss of symmetry in the molecular arrangement and thus prevents the generation of any measurable signal. We probed our films instead by dielectric spectroscopy to gain information about the degree of correlation in the molecular orientation, that is the BOO. After depositing our films in the glassy state, we monitored their dielectric response during annealing above T g , which permitted the measurement of their dielectric strength Δ ε , that is, the contribution of the orientational polarization to the dielectric constant (see below). This quantity is a robust parameter for measuring the BOO, as it is sensitive to the orientation correlation among neighbouring dipoles, via the Kirkwood factor g . Indeed, Δ ε ≈ g < μ 2 >/ k B T (ref. 27 ), where μ is the molecular dipole moment and g accounts for the correlation among neighbour molecular dipole moments. The value of g is given by where z is the number of correlated molecules around a given central molecule, and <cos ψ > is a statistically averaged cosine of the angle ψ between two neighbouring dipoles. Thus, if the dipoles have a tendency for parallel orientation, then g >1, whereas 0< g <1 implies an antiparallel orientation. A random orientation of the dipoles, instead, results in g =1. Accordingly, if an enrichment in MRO regions is finally obtained, the orientational correlation is locally enhanced, leading to an increase or a decrease in the value of g , depending on the spatial organization of the molecules in the local clusters. We anticipate that in the specific case of our investigation, we found a clear enhancement of Δ ε and a consequent increase in g , indicating a parallel orientational correlation among the dipoles, which can be justified by the presence of (locally preferred) anisotropic structures. Moreover, such an increase rules out the presence of long-range order and crystal-like BOO, which would instead cause a decrease in the dielectric response due to the suppression of the rotational and translational modes in these clusters. Furthermore, as a consequence of a larger correlation length, the MRO regions are expected to have slower structural dynamics (corresponding to ~2–10 τ ) with respect to the isotropic liquid [28] , [29] . Dielectric response of a liquid with enhanced BOO In glycerol films (~10–130 nm), we found a tremendous enhancement in the dielectric strength ( Fig. 1 ), exceeding by more than threefold the value measured for bulk glycerol films deposited well above T g (ref. 30 ). Such a large value cannot be rationalized by a mere increase in density, which would prompt non-physical changes, nor by a larger effective dipole moment, due to a very unlikely perfectly planar orientation in the direction of the electric field. We ascribe this increase to a higher orientational correlation among the dipole moments, which is consistent with the concept of a liquid state having enhanced MRO and BOO, compared with the OL. Hereafter, this particular liquid phase will be denoted as medium-range order enriched liquid (MROL). 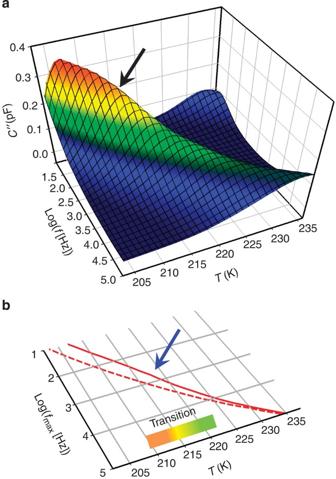Figure 1:Temperature and frequency dependence of the dielectric response. Evolution of the dielectric response in an 11-nm-thick glycerol film of vapour deposited at 166 K (0.88Tg). (a) The temperature dependence ofC″(f,T), the imaginary part of the capacitance, presents a strong, gradual reduction in the intensity of the structural peak observed atT>203 K. (b) The frequencyfmax, corresponds to the maximum of the relaxation peak in the curveC″ versus log(f) and is related to the structural relaxation time, via the relationshipτ=1/(2πfmax). This quantity is given as a function of temperature for the metastable highly ordered liquid (solid line) and compared with the values obtained for bulk glycerol (dashed line). These last values are in excellent agreement with the values obtained from measurements performed after cooling. The arrows indicate the onset of the transition. Figure 1: Temperature and frequency dependence of the dielectric response. Evolution of the dielectric response in an 11-nm-thick glycerol film of vapour deposited at 166 K (0.88 T g ). ( a ) The temperature dependence of C ″( f , T ), the imaginary part of the capacitance, presents a strong, gradual reduction in the intensity of the structural peak observed at T >203 K. ( b ) The frequency f max , corresponds to the maximum of the relaxation peak in the curve C ″ versus log( f ) and is related to the structural relaxation time, via the relationship τ =1/(2 πf max ). This quantity is given as a function of temperature for the metastable highly ordered liquid (solid line) and compared with the values obtained for bulk glycerol (dashed line). These last values are in excellent agreement with the values obtained from measurements performed after cooling. The arrows indicate the onset of the transition. Full size image Concurrently, we observed structural relaxation times 4–5-fold longer than the relaxation time of the OL, corresponding to a shift in T g of ~4 K. This finding is in line with the quantitative predictions proposed both for Lennard–Jones liquids [28] and for model polymeric systems [29] . To quantify the perturbation in the molecular orientation in the MROL, we analysed the temperature evolution of Δ ε N =Δ ε MROL /Δ ε OL . The isothermal dielectric spectra acquired upon annealing showed that Δ ε N begins to decrease at an onset temperature depending on the material, on the thickness of the films and on the temperature of deposition ( Figs 2 and 3 ), which indicates the metastable nature of the ordered structures. We were able to observe the MROL→OL transition via the temperature evolution of Δ ε N ( Fig. 2 , Methods and Supplementary Fig. S1 ). The OL behaviour, that is, Δ ε N =1, is eventually recovered after prolonged annealing at T > T g . It must be noted that, compared with Δ ε , τ is a less sensitive parameter to the presence of MRO. The variation of Δ ε with the concentration of MRO regions is remarkably larger with respect to the evolution of τ , which allows a better resolution in monitoring the MROL→OL transition ( Supplementary Fig. S2 ). 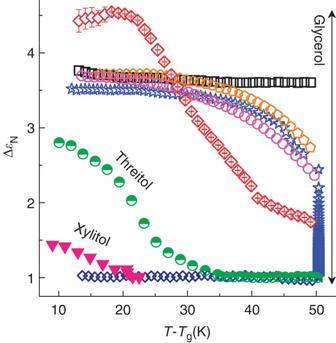Figure 2:Values of the dielectric strength. Values are normalized to those in the ordinary supercooled liquid (ΔεN=Δε/ΔεOL). The figure shows the temperature evolution of ΔεNat different thicknesses and for different polyols. Changes in ΔεNfor glycerol films (open symbols) of different thicknesses, evaporated at 0.88Tg(red diamonds, 11 nm; purple circles, 25 nm; open orange pentagons, 50 nm; open black squares, 126 nm). Values of ΔεNfor a 65-nm-thick film of threitol (semi-open green circles) and a 65-nm-thick film of xylitol (pink triangles) evaporated at 0.88Tg, are added for comparison: a similar enhancement of Δεis observed for these materials, albeit to a minor extent and with minor stability. The open blue stars represent the values of ΔεNfor the heating scans of an 89-nm-thick glycerol film deposited at 0.97Tg, successively held at 238 K for 23 h. Open navy diamonds are the literature data for a 27-nm film deposited aboveTg(ref.30). Error bars take into account the uncertainties in the determination of the dielectric strength via the fitting procedure described in theMethodssection. If not explicitly indicated, error bars are smaller than the symbol size. Figure 2: Values of the dielectric strength. Values are normalized to those in the ordinary supercooled liquid (Δ ε N =Δ ε /Δ ε OL ). The figure shows the temperature evolution of Δ ε N at different thicknesses and for different polyols. Changes in Δ ε N for glycerol films (open symbols) of different thicknesses, evaporated at 0.88 T g (red diamonds, 11 nm; purple circles, 25 nm; open orange pentagons, 50 nm; open black squares, 126 nm). Values of Δ ε N for a 65-nm-thick film of threitol (semi-open green circles) and a 65-nm-thick film of xylitol (pink triangles) evaporated at 0.88 T g , are added for comparison: a similar enhancement of Δ ε is observed for these materials, albeit to a minor extent and with minor stability. The open blue stars represent the values of Δ ε N for the heating scans of an 89-nm-thick glycerol film deposited at 0.97 T g , successively held at 238 K for 23 h. Open navy diamonds are the literature data for a 27-nm film deposited above T g (ref. 30 ). Error bars take into account the uncertainties in the determination of the dielectric strength via the fitting procedure described in the Methods section. If not explicitly indicated, error bars are smaller than the symbol size. 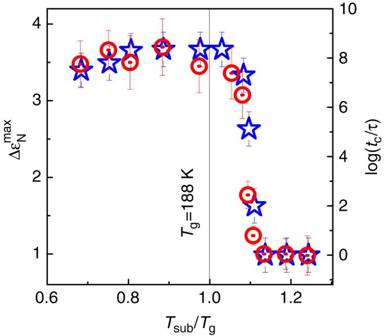Figure 3:Effect of substrate temperature during deposition on the enhancement of dielectric response and on stability of the medium-range order enriched liquid. The blue stars represent the maximum enhancement in the dielectric strength, ΔεNmax, as a function of the temperature of the substrateTsubduring deposition; the red centred circles indicate the conversion timetcfrom the MROL to OL phases, normalized by the relaxation timeτ, for 30-nm-thick glycerol films. The value oftchas been evaluated as the elapsed time after which a 30-nm-thick film is 15% converted into the OL phase. Error bars are related to the determination of the structural relaxation time and of the dielectric strength via the fitting procedure described in theMethodssection. Full size image Figure 3: Effect of substrate temperature during deposition on the enhancement of dielectric response and on stability of the medium-range order enriched liquid. The blue stars represent the maximum enhancement in the dielectric strength, Δ ε N max , as a function of the temperature of the substrate T sub during deposition; the red centred circles indicate the conversion time t c from the MROL to OL phases, normalized by the relaxation time τ , for 30-nm-thick glycerol films. The value of t c has been evaluated as the elapsed time after which a 30-nm-thick film is 15% converted into the OL phase. Error bars are related to the determination of the structural relaxation time and of the dielectric strength via the fitting procedure described in the Methods section. Full size image Similar perturbations to the dielectric function have been observed for natural rubber, following the application of a tensile stress: although the value of Δ ε tripled, τ remained unaffected by stretching [31] . In glycerol films (thicker than 20 nm), we observed an enhancement by a factor of 3.7 in Δ ε N and a simultaneous increase of 4.5-fold in the relaxation time; during the MROL→OL transition, these alterations led to a broadening of the relaxation peak in the dielectric loss, without separation between the contributions from the MRO regions and from the amorphous liquid ( Supplementary Figs S1 and S3 ). For these reasons, we concentrated our investigation mainly on the dielectric strength. Additional experiments on larger homologous molecules, such as threitol and xylitol, revealed the same trends as for glycerol, but to a lesser extent (smaller Δ ε N and lower onset temperatures, Fig. 2 ), which further supports the H-bonding interaction as the origin of the enhanced orientational correlation. Indeed, the larger multiplicity of molecular conformations that arise from the higher intramolecular degrees of freedom with increasing molecular size, likely reduces the efficiency of the formation of an ordered intermolecular network. Such a trend is in further agreement with the idea that the more fragile glass formers ( m xylitol > m threitol > m glycerol , (ref. 32 ) with m the fragility) are characterized by lower frustration, that is, by a lower concentration of (locally) ordered structures [11] , [28] , which explains the smaller increase in polarization with increasing molecular size. Lifetime and length scale of the enhancement in polarization We gained further insight into the origin of the MRO regions and the related increase in Δ ε of the MROL phase by investigating the dielectric response of 30-nm-thick glycerol films, grown holding the substrate at different temperatures, T sub . After deposition, we measured Δ ε N during identical temperature scans, and we analysed the impact of T sub on the maximum value of the increase in dielectric strengths, Δ ε N max , as observed before the onset of the transition to the OL ( Fig. 3 , red circles). To relate this parameter to the kinetic stability of the MROL phase, we compared its temperature dependence with the temperature dependence of the conversion time t c normalized to the value of τ at the same temperature (blue stars). The excellent match between the trends of these two quantities proves that an enhancement in dielectric strength, that is, a higher orientational order, is correlated with a greater stability of the MROL phase. The normalized dielectric strength and the value of log( t c / τ ) remained almost constant up to T sub =206 K, where an abrupt simultaneous drop in both parameters took place. Within the limits of our experimental method, we observed no enhancement in Δ ε N for films deposited at T sub ≥213 K, which determined the limiting temperature where we could detect a deviation from the OL. This behaviour suggests the onset of the stability of a liquid phase with enhanced orientational order below T *~213 K (< T m ). We conducted further experiments that verified that the increase in the dielectric susceptibility of the metastable liquid state also varies with the film thickness ( Fig. 4 ). The increase in Δ ε N exceeds 5.0 at 9 nm, and Δ ε N max decays progressively before settling to a constant value of 3.7, in films thicker than 15–20 nm. Given the purely additive contribution of each layer to the dielectric strength in our experimental configuration [33] , we might imagine a higher BOO in proximity to the interfaces, penetrating for a few nanometres. Such a length scale is larger than has been observed in metallic liquids in proximity to the crystal growth front [34] , where only a few atomic layers are affected. We were able to fit the interfacial excess in Δ ε N with a single exponential with a characteristic decay length of 5.9±1.0 nm. This value can be treated as an upper bound for the actual spatial extent of the extra BOO in proximity to the substrate, and thus also for the size of the region where the liquid dynamics is affected by the MRO [35] . 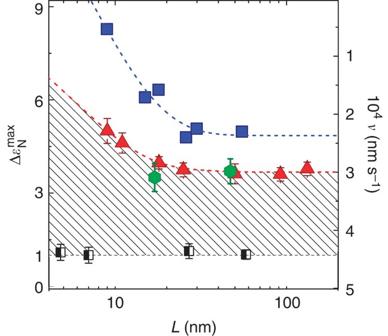Figure 4:Comparison between maximum enhancement in dielectric strength and conversion rate to the ordinary liquid phase. Thickness dependence of the maximum enhancement in dielectric strength, ΔεNmax, determined atTg+20 K, before the onset of the conversion into the OL phase (red triangles). This quantity is a measurement of the glassy structural order. Green hexagons refer to MROL glycerol films grown on top of a layer previously deposited aboveTg. The semi-open black squares represent the literature data on glycerol films deposited aboveTg(ref.30). The blue squares indicate the transformation ratevatTg+45 K, please note that the righty-axis goes from the top to the bottom. The dotted red and the blue lines represent the exponential fits of the thickness dependence of ΔεNmaxand ofv; characteristic decay lengths of 5.9±1.0 nm and 7.2±2.0 nm were obtained, respectively. For comparison to the trend shown inFig. 2and a detailed description of the calculation of ΔεNand the conversion timetc, see theSupplementary Methods. Error bars are related to the determination of the dielectric strength via the fitting procedure described in theMethodssection. Figure 4: Comparison between maximum enhancement in dielectric strength and conversion rate to the ordinary liquid phase. Thickness dependence of the maximum enhancement in dielectric strength, Δ ε N max , determined at T g +20 K, before the onset of the conversion into the OL phase (red triangles). This quantity is a measurement of the glassy structural order. Green hexagons refer to MROL glycerol films grown on top of a layer previously deposited above T g . The semi-open black squares represent the literature data on glycerol films deposited above T g (ref. 30 ). The blue squares indicate the transformation rate v at T g +45 K, please note that the right y -axis goes from the top to the bottom. The dotted red and the blue lines represent the exponential fits of the thickness dependence of Δ ε N max and of v ; characteristic decay lengths of 5.9±1.0 nm and 7.2±2.0 nm were obtained, respectively. For comparison to the trend shown in Fig. 2 and a detailed description of the calculation of Δ ε N and the conversion time t c , see the Supplementary Methods . Error bars are related to the determination of the dielectric strength via the fitting procedure described in the Methods section. Full size image To discern the impact of the interface-induced ordering caused by steric effects from the possible impact of molecular interactions with the substrate [36] , we investigated MROL glycerol films grown on OL layers of the same material, previously deposited well above T g (see Supplementary Methods for further details). We obtained quantitative agreement with the values measured in the single-layer films of comparable thickness, proving that the interactions between the polyols and the substrate of the interdigitated electrodes (IDE) do not influence the structure of the MROL phase. To further analyse the transformation process, we prepared glycerol films with different thicknesses, and we estimated the velocity v of the conversion of the MROL into the OL by analysing the isothermal decay in Δ ε N at increasing annealing temperatures. We found conversion rates on the order of 10 −4 nm s −1 at T g +50 K for films thicker than 15 nm, while below this threshold, v increases exponentially, with a characteristic length of (7.2±2.0) nm, similar to the value found for Δ ε N max ( Fig. 4 ). The outcome of this experiment, in which we kept T sub constant and we varied the layer thickness, is in line with the data in Fig. 3 , relative to measurements where we evaluated the conversion time at constant thickness, but at different T sub . Such behaviour, with the temperature dependence observed for films of larger homologous molecules ( Fig. 2 ), provides a further confirmation that higher values of Δ ε N correspond to a greater kinetic stability of the MROL. Moreover, the linear decay of Δ ε N during isothermal transformation, indicating a constant transformation rate, is consistent with the scenario of a growth front-like transformation process where the liquid–liquid interface between the two phases propagates through the film at a constant velocity, inversely proportional to the increase in orientational polarization of the structural process in the liquid state [37] . Further investigations will be necessary to unveil the molecular origin of the transformation process and the origin of such high kinetic stability. A rationalization of the observed values of t c / τ would require determining the lifetime of the LPSs and their stability against annealing. The MRO enrichment should persist as long as the LPSs have not recovered their equilibrium concentration at a given temperature. Until the achievement of this condition, the MRO regions continuously destroy and nucleate, driven by the minimization of local free energy, achieved via spatial reorganization at the time scale of τ (refs 11 , 28 ). This long-lasting behaviour permitted us to detect the differences in the orientational polarization. At present, no simulation methods are available to compute the distribution and the exact lifetime of these metastable structures, even using state-of-the-art computer resources [11] . However, recent Monte Carlo simulations have verified that metastable states associated with lower inherent structure energy (that is, LPSs) can survive for lifetimes longer than the lifetimes predicted by simple diffusion models and can thus coexist with the isotropic liquid [38] . We speculate that our preparation method permitted us to obtain similar long-lived structures, ensuring the persistence of the enhanced MRO in our systems. This success was possible because, as anticipated, performing PVD below T g has been proven to be the most efficient way to age glasses. In the supporting information, we analyse the similarities between the results from our experiment and previous investigations of ordinary and ultrastable glasses ( Supplementary Figs S4–S6 ). Because of the importance of such domains in determining the properties of the glass transition, we believe that the procedure described in this work, which allows the preparation of isotropic liquids enriched in conformations present in the glassy state, represents a possible method of achieving hidden liquid phases with intriguing materials properties. We hope that our work will stimulate further investigation of this new liquid phase via different experimental approaches, which will make it possible to test theoretical models to clarify the nature of the glass transition. Molecular beam deposition in the glassy state Films of glycerol, threitol and xylitol (degree of purity >99%, purchased from Aldrich), were prepared by organic molecular beam deposition directly on the IDE [30] , [39] , [40] , which made it possible to probe their dielectric response. The bulk material was heated above its melting temperature in a crucible connected, via a pneumatic valve, to a vacuum chamber maintained at a pressure p ~10 –8 mbar. The thickness of the films, monitored via a quartz crystal microbalance (QCM), was varied by switching the valve; the temperature of the crucible was adjusted to keep the evaporation rate below 3 × 10 −2 nm s −1 . During evaporation, the temperature of the substrate, T sub , was maintained at 0.88 T g ; this value was very close to the temperature providing the best thermal and kinetic stability of the MROL, as indicated by additional experiments performed on 50-nm-thick glycerol films grown at different T sub in the range from 0.75 T g to T g . To prepare the glycerol bilayers, layers of different thickness (6 and 36 nm) were deposited at 223 K (1.2 T g ) and immediately after deposition cooled to 0.88 T g , where the evaporation of an 11-nm capping layer followed the same protocol used for the single layers. Dielectric measurements To perform in situ dielectric spectroscopy while permitting a continuous evaporation of material on the target substrate, we employed IDE structures, which present an open-electrode configuration. The sensors, produced by UV lithography, were composed of 100 gold fingers (height=200 nm; width=15 μm) deposited on a quartz substrate. Each pair of fingers is spaced 1.25 μm apart, resulting in a total capacitance of 5 pF. Silver wires were glued on the connectors of the IDE via a thermally and electrically conductive epoxy resin filled with silver nanoparticles (Ecolit E 325) and soldered to a high-vacuum feedthrough, which allowed connection to an impedance analyser (ALPHA, Novocontrol). The intensity of the applied electric field E was <10 6 V m −1 , a regime in which the polarization response is linearly proportional to E . The IDE was mechanically attached to a metallic plate located inside the vacuum chamber and held at the desired temperature by the combined action of a resistance heating and a cooling flux of gaseous nitrogen. A Pt100 sensor was glued to the substrate of the IDE with Elecolit E 325 to constantly monitor T sub . In addition to the direct QCM measurements, the thickness of the film could also be checked based on the dielectric signal, according to the equation Δ C ∞ = N ε 0 ( ε ∞ −1)( p / d ) L , where L is the thickness of the film; Δ C ∞ is the resulting change in the capacitance of the system; ε 0 is the vacuum permittivity; ε ∞ is the dielectric constant of the material; N is the total number of fingers; and p and d indicate the length of the fingers of the IDE and their mutual distance, respectively. Such a procedure was used below 30 nm, where the error in determining the thickness by QCM, due to the different position of the two sensors, exceeded 10%. The measured increase of the dielectric strength is a strong proof of the lack of bubbles inside our films, which, acting as dielectric cavities ( ε ∞ vacuum < ε ∞ glycerol ) would reduce the polarization and thus the dielectric signal. Characterization of the MROL phase After deposition, the films were heated to a temperature T = T g +10 K and subsequently annealed up to T g +50 K in steps of 1 K. Isothermal dielectric spectra were acquired at each temperature, in the frequency range between 10 −1 and 10 6 Hz. The values of the relaxation time τ were derived from the relation τ =2 π / f max , where f max is the frequency at which the imaginary part of the dielectric permittivity ε ″( ω ) shows a maximum. The values of the dielectric strength were obtained by analysing the isothermal spectra via the empirical Havriliak–Negami (HN) function: where Δ ε , τ HN , α , and β are the dielectric strength, the relaxation time and the shape parameters, respectively, accounting for the width and the asymmetry of the loss curves. Further isothermal measurements were performed on glycerol films of different thicknesses (9, 15, 18, 26, 30, 55, 89 nm): the temperature of the IDE was varied in the same range as above, but in steps of 5 K. The sample was held at each annealing temperature for 2 h. The conversion rate into the OL phase, v , was estimated by fitting isothermal scans with linear decays v =Δ l /( t − t 0 ), where Δ l is the fraction of transformed film, and t 0 indicates the onset of measurement. The value of Δ l is obtained from the time evolution of the dielectric strength under the assumption that Δ ε is the sum of the contribution of the two liquid phases averaged over their volume fractions according to Δ ε TOT = x OL · R Δ ε OL + x MROL Δ ε OL = R Δ ε OL ( L −Δ l )/ L +Δ ε OL ·Δ l / L , where x is the volume fraction, R =Δ ε N max /Δ ε OL . The dielectric strength of the film normalized by the value in the OL, Δ ε OL , is thus given by Δ ε N ( t − t 0 )=Δ ε TOT ( t − t 0 )/(Δ ε OL · L )= R −( R −1)·Δ l / L , which simplifies to Δ ε N ( t 0 )−Δ ε N ( t − t 0 )=( R −1)·Δ l / L . Finally, v = L/ ( t − t 0 )·[Δ ε N ( t 0 )−Δ ε N ( t − t 0 )]/( R −1). We ruled out the possibility that the larger values of Δ ε and of τ observed in the medium-range crystalline order phase are actually induced by the presence of water or other contamination in the films. Water molecules would instead enhance the structural relaxation time (plasticizing effect) and reduce the dielectric strength by breaking the OH bonds. [41] , [42] Contamination by other impurities would also break the intermolecular OH bonds, whose fluctuations contribute to the Δ ε of polyols, and consequently reduce the dielectric strength. Furthermore, we considered whether the observed enhancement in the dielectric strength and its thermal evolution could be due to the presence of ionic impurities intruded into the films during deposition, and subsequently desorbing at higher temperatures, during annealing. Such a mechanism could mimic the conversion of the MROL phase into the OL. In addition to increase in the value of the dielectric strength, ionic contaminants would, in fact, also yield a larger conductivity σ , see Supplementary Methods and Supplementary Equation S2 . To verify the validity of this conjecture, we performed isothermal experiments at 228 K, a temperature high enough to simultaneously observe the evolution of the dielectric strength and of the conductivity. The results ( Supplementary Fig. S7 ) show that the dielectric strength decays linearly with the annealing time, whereas the conductivity remains at a constant value, comparable with that of films deposited at T » T g . This evidence strongly excludes the possibility that the observed enhancement in dielectric strength is due to the presence of contaminants. How to cite this article: Capponi, S. et al. Supercooled liquids with enhanced orientational order. Nat. Commun. 3:1233 doi: 10.1038/ncomms2228 (2012).